Chirality-controlled synthesis of single-wall carbon nanotubes using vapour-phase epitaxy Chirality-controlled synthesis of single-wall carbon nanotubes with predefined chiralities has been an important but elusive goal for almost two decades. Here we demonstrate a general strategy for producing carbon nanotubes with predefined chiralities by using purified single-chirality nanotubes as seeds for subsequent metal catalyst free growth, resembling vapour-phase epitaxy commonly used for semiconductor films. In particular, we have successfully synthesized (7, 6), (6, 5) and (7, 7) nanotubes, and used Raman spectroscopy to show unambiguously that the original chiralities of the nanotube seeds are preserved. Furthermore, we have performed electrical measurements on synthesized individual (7, 6) and (6, 5) nanotubes, confirming their semiconducting nature. The vapour-phase epitaxy approach is found to be highly robust and should enable a wide range of fundamental studies and technological developments. Single-wall carbon nanotubes (SWCNTs) possess superior electrical and optical properties, and hold great promise for electronic and biomedical applications [1] , [2] , [3] , [4] , [5] , [6] , [7] , [8] , [9] , [10] . As the electronic property of an SWCNT strongly depends on its chirality, the lack of synthetic control in chirality has long been recognized as a fundamental impediment in the science and application of SWCNTs. Previous efforts to address this issue have resulted in significant progress in separation of synthetic mixtures, yielding predominantly single-chirality nanotube species [11] , [12] , [13] , [14] , [15] . However, separation processes are limited by their small scale, high cost and short length (<500 nm) of the resulting chirality-pure nanotubes. They are, therefore, not suitable for many, especially electronic device applications. Realistic application of SWCNTs in electronic devices and integrated circuits requires that the electronic type of the nanotubes be well controlled. Selective synthesis of semiconducting or metallic predominated SWCNTs has already been achieved through controlled chemical vapour deposition (CVD) growth [16] , [17] , [18] , enabling the fabrication of nanotube field-effect transistors using predominantly semiconducting SWCNTs [19] , [20] . As a next step, synthesis of SWCNTs with predefined chirality is highly desired. However, this goal has remained elusive for some time in the nanotube field. For metal-catalysed nanotube synthesis by CVD, it is generally believed that the diameters of the nanotubes are determined by the size of the catalytic metal particles. Unfortunately, attempts to control the size of the catalysts in hope of achieving chirality-controlled nanotube growth have not been successful [21] . Nanotube ‘cloning’ has been studied with [22] , [23] and without [24] metal catalyst particles showing various degree of success; however, controlled synthesis of nanotubes with predefined chiralities has not been achieved. In contrast, vapour-phase epitaxy (VPE) such as molecular beam epitaxy and metal organic CVD has long been used by the semiconductor industry to grow two-dimensional epitaxial films, which can preserve the crystalline structure of the starting substrate. It is, therefore, very intriguing to explore the potential of using VPE for one-dimensional nanotube synthesis. Here we demonstrate a VPE-analogous general strategy for producing nanotubes of predefined chirality. Our strategy is to combine nanotube separation with synthesis to achieve controlled growth of nanotubes with preselected chirality. Tremendous progress has been made in recent years in SWCNT separation [11] , [12] , [13] , [14] , [15] , [25] , [26] . In particular, DNA-based chromatographic separation allows purification of both semiconducting and metallic single-chirality SWCNTs through the use of different DNA sequences [12] , [26] . In this work, three exemplary chirality-pure (7, 6), (6, 5) and (7, 7) SWCNT seeds with purity up to 90% are used. These serve as the starting templates for the ensuing catalyst-free, chirality-controlled nanotube cloning process. We show that purified single-chirality nanotube seeds of both semiconducting and metallic SWCNTs are significantly elongated through a catalyst-free VPE process, producing horizontally aligned SWCNT arrays on quartz substrates and randomly oriented SWCNTs on Si/SiO 2 substrates, with lengths more than tens of micrometres. Raman characterization confirms that the original chiralities of the nanotube seeds are preserved in the extended portion of the nanotubes, and the semiconducting nature of the grown (7, 6) and (6, 5) SWCNTs are further confirmed using electrical measurements on individual nanotubes. Deposition and activation of chirality-pure nanotube seeds The schematic of the chirality-controlled SWCNTs cloning process is illustrated in Fig. 1 (see Methods for details). First, chirality-pure SWCNT seeds obtained from the DNA-based separation were deposited onto the growth substrates using drop coating and incubation with different durations (see Methods ). The as-deposited seeds then went through an air and water vapour annealing process. This step removes the DNA wrapped on the nanotube seeds and activates the nanotube ends so that carbon reaction intermediates from decomposed feed stock can be efficiently added. Both methane and ethanol were found to be suitable as the carbon feed source to achieve chirality-controlled growth from these seeds. 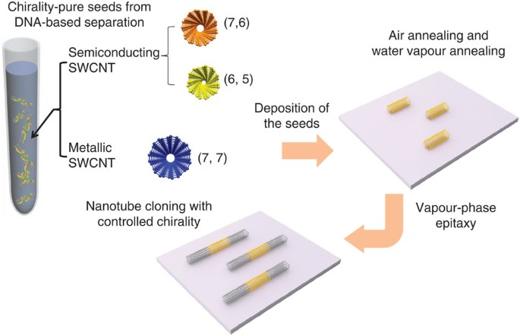Figure 1: Schematic illustration of the VPE process for chirality-controlled SWCNT synthesis. The chirality-pure nanotube seeds obtained from DNA-based separation are first deposited onto various kinds of substrates, including quartz and Si/SiO2, followed by air annealing and water vapour annealing processes to activate the ends for the ensuing VPE growth. VPE with either methane or ethanol as the carbon feed stock is then used to achieve chirality-controlled growth from these seeds. Figure 1: Schematic illustration of the VPE process for chirality-controlled SWCNT synthesis. The chirality-pure nanotube seeds obtained from DNA-based separation are first deposited onto various kinds of substrates, including quartz and Si/SiO 2 , followed by air annealing and water vapour annealing processes to activate the ends for the ensuing VPE growth. VPE with either methane or ethanol as the carbon feed stock is then used to achieve chirality-controlled growth from these seeds. Full size image A critical factor that determines the yield of the VPE cloning process is the air and water vapour annealing process. This was revealed by a systematic study we performed to map out the optimum annealing conditions. As shown in the Supplementary Information ( Supplementary Fig. S1 ), without proper annealing treatment, the cloning yield is extremely low, with only curvy nanotube bundles visible after growth. In comparison, after a proper air and water vapour annealing, individually dispersed, long and straight nanotubes can be grown. We speculate that the air and water annealing processes alter functional groups on nanotube ends, such that the ends are activated and capable of incorporating incoming carbon atoms for growth. We note that the nanotube seeds are very sensitive to the annealing environment, and 30–50% of seeds were etched away during the air and water annealing processes ( Supplementary Fig. S2 ). Extensive studies to compare the VPE cloning results obtained with different temperatures and duration of the annealing steps, as well as gas flow rates ( Supplementary Table S1 and Supplementary Fig. S3 ), led to an optimum recipe described in the Methods section. Characterization of cloned nanotubes using microscopy We used atomic force microscopy (AFM) and scanning electron microscopy (SEM) to characterize SWCNTs before and after VPE cloning. Representative AFM images of (7, 6) SWCNT before and after cloning using ethanol on quartz substrates are presented in Fig. 2a , respectively. The average length of the nanotubes after cloning was measured to be 34.5±17.7 μm ( Fig. 2d ), significantly longer than the average length of 0.34±0.15 μm for the as-purified (7, 6) nanotube seeds ( Fig. 2c ). The measured diameter of the cloned nanotubes were approximately 0.9 nm, consistent with the (7, 6) nanotube diameter ( d =0.89 nm). As control experiments, blank quartz substrates and quartz substrates deposited with DNA solution but without any nanotube seeds were subjected to the air and water vapour annealing, and then the VPE cloning. No nanotube growth was observed after the VPE process ( Supplementary Figs S5 and S6 ). This demonstrates that the long SWCNTs were indeed grown from the nanotube seeds. 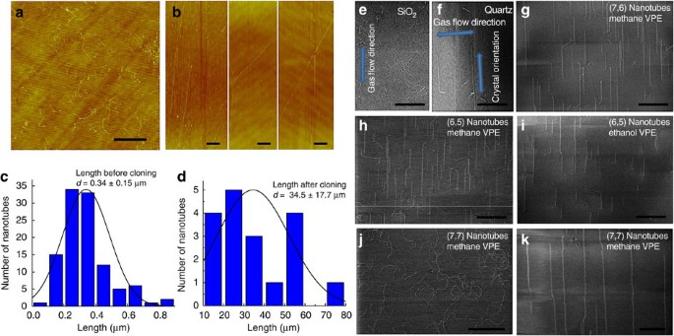Figure 2: AFM and SEM characterization of SWCNTs before and after VPE. (a,b) AFM images of (7, 6) nanotubes before and after VPE using ethanol on quartz substrates. The scale bars in a and b are 1 μm. (c,d) Length distribution of the (7, 6) nanotubes before and after VPE. (e,f) Comparison of (7, 6) nanotubes cloned on quartz and Si/SiO2substrates. (g) An SEM image showing (7, 6) nanotubes cloned on the quartz substrate using methane. (h,i) SEM images of (6, 5) nanotubes cloned on quartz substrates using methane and ethanol, respectively. (j,k) SEM images of (7, 7) nanotube cloned on quartz and Si/SiO2substrates. Scales bars, 50 μm for (e,f) andj, 30 μm for (g,h) andi, and 10 μm fork. Figure 2: AFM and SEM characterization of SWCNTs before and after VPE. ( a , b ) AFM images of (7, 6) nanotubes before and after VPE using ethanol on quartz substrates. The scale bars in a and b are 1 μm. ( c , d ) Length distribution of the (7, 6) nanotubes before and after VPE. ( e , f ) Comparison of (7, 6) nanotubes cloned on quartz and Si/SiO 2 substrates. ( g ) An SEM image showing (7, 6) nanotubes cloned on the quartz substrate using methane. ( h , i ) SEM images of (6, 5) nanotubes cloned on quartz substrates using methane and ethanol, respectively. ( j , k ) SEM images of (7, 7) nanotube cloned on quartz and Si/SiO 2 substrates. Scales bars, 50 μm for ( e , f ) and j , 30 μm for ( g , h ) and i , and 10 μm for k . Full size image We also carefully studied the effect of substrates on the VPE cloning process. On Si/SiO 2 substrates ( Fig. 2e ), random orientation was observed for the cloned nanotubes irrespective of the gas flow direction. For nanotube cloning performed on the ST-cut quartz substrates ( Fig. 2f ), the cloned SWCNTs were found to be horizontally aligned along the crystal orientation [27] . This should be very useful for the fabrication of nanotube transistors and integrated circuits. Overall, the nanotube VPE process was found to be very robust and highly reproducible. Various carbon feed stocks including methane and ethanol, and different nanotube seeds including (7, 6), (6, 5) and (7, 7) were used successfully. The SEM images of (7, 6) nanotubes cloned with methane ( Fig. 2g ), (6, 5) nanotubes cloned with methane ( Fig. 2h ) and ethanol ( Fig. 2i ), respectively, indicate that similar growth were achieved for all the cases. VPE cloning process is also demonstrated for the (7, 7) armchair metallic nanotube using both Si/SiO 2 ( Fig. 2j ) and quartz ( Fig. 2k ) as substrate. Chirality identification by Raman spectroscopy To determine whether the original chiralities were preserved during the cloning process, we used micro-Raman to characterize the pristine and cloned SWCNTs. For the (7, 6) case, we used 1.96 eV laser excitation, which is close to the second optical transition E 22 =1.92 eV of the (7, 6) nanotubes [28] . To further enhance the signal-to-noise ratio, surface-enhanced Raman spectroscopy was used after e-beam evaporation of 5 nm silver on the substrate ( Supplementary Fig. S8 ). The radial breathing mode (RBM) Raman spectra taken at different random locations on the substrates before and after cloning are presented in Fig. 3a , respectively. For small diameter nanotubes such as (7, 6), (6, 5) and (7, 7), adjacent nanotubes have very distinct RBM frequencies ( Fig. 3f ) [29] , allowing unambiguous chirality assignment by determining the RBM frequency and the laser excitation energy. 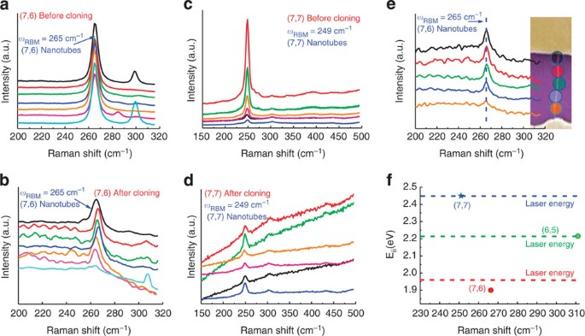Figure 3: Raman spectroscopy characterization of SWCNTs before and after VPE. (a,b) Raman RBMs of (7, 6) nanotubes before and after VPE. The spectra were taken at different random locations on the quartz substrates with laser excitation energy of 1.96 eV. The peaks at 265 cm−1correspond to the RBM of (7, 6) nanotubes. (c,d) Raman RBMs of (7, 7) nanotubes before and after VPE. The spectra were taken at different random locations on the Si/SiO2substrates with laser excitation energy of 2.4 eV. The peaks at 249 cm−1correspond to the RBM of (7, 7) nanotubes. (e) Raman RBM spectra along a specific nanotube confirming that the chirality is preserved after the VPE process. Inset, an SEM image (with artificial colour) of the nanotube. (f) Kataura plot shows the RBM frequencies andEiiof different nanotubes. The values were taken from the literature29. Figure 3a show predominant peaks at 265 cm −1 , which correspond to the RBM of (7, 6) nanotubes, indicating that the chirality is indeed preserved in the cloned nanotubes. The minority peaks at 300 and 307 cm −1 can be attributed to the (8, 3) and (9, 1) impurities. We have also performed Raman mapping along a specific nanotube as shown in Fig. 3e , confirming that the chirality is preserved along the whole nanotube. Similar studies were carried out for (7, 7) nanotubes using 2.4 eV laser excitation; Raman spectra of (7, 7) before ( Fig. 3c ) and after VPE growth ( Fig. 3d ) showed predominant peaks at 249 cm −1 , which correspond to the RBM of (7, 7) nanotubes. The weak peak at 303 cm −1 is attributed to the Si/SiO 2 substrate background. The RBM intensity of cloned nanotubes is weaker than that of the nanotube seeds. This is because many nanotube seeds got etched away during the annealing and subsequent VPE step, thus leading to reduced nanotube number density and reduced Raman intensity. Figure 3: Raman spectroscopy characterization of SWCNTs before and after VPE. ( a , b ) Raman RBMs of (7, 6) nanotubes before and after VPE. The spectra were taken at different random locations on the quartz substrates with laser excitation energy of 1.96 eV. The peaks at 265 cm −1 correspond to the RBM of (7, 6) nanotubes. ( c , d ) Raman RBMs of (7, 7) nanotubes before and after VPE. The spectra were taken at different random locations on the Si/SiO 2 substrates with laser excitation energy of 2.4 eV. The peaks at 249 cm −1 correspond to the RBM of (7, 7) nanotubes. ( e ) Raman RBM spectra along a specific nanotube confirming that the chirality is preserved after the VPE process. Inset, an SEM image (with artificial colour) of the nanotube. ( f ) Kataura plot shows the RBM frequencies and E ii of different nanotubes. The values were taken from the literature [29] . Full size image Electron transport measurement of cloned nanotubes Back-gated nanotube field-effect transistors were fabricated to further characterize the electrical properties of the cloned (7, 6) and (6, 5) nanotubes. The device schematic and an SEM image of a representative device consisting of an individual (7, 6) nanotube are shown in Fig. 4a , respectively. In brief, the cloned (7, 6) nanotubes grown on quartz substrates were transferred to Si/SiO 2 substrates with 50 nm SiO 2 using methods described in our previous publication [9] . This was followed by formation of Ti/Pd (0.5/50 nm) source/drain metal contacts using lithography and lift-off techniques. After production, the device had a channel length of L =4 μm and a 50-nm-thick SiO 2 gate dielectric. 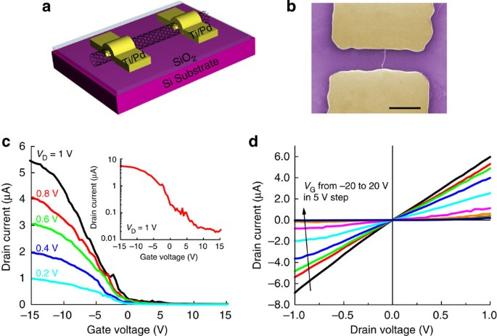Figure 4: Electrical characterization of the cloned (7, 6) SWCNTs. (a) Schematic and (b) an SEM image (with artificial colour) of a back-gated (7, 6) nanotube transistor. The device consists of an individual (7, 6) nanotube, withL=4 μm and 50 nm thick SiO2gate dielectric. Scale bar, 5 μm forb. (c) Transfer characteristics (ID–VG) of the transistor measured at variousVDbiases. Inset, transfer characteristics plotted in semi-logarithm scale withVD=1 V. (d) Output (ID–VD) characteristics of the same device measured at variousVGbiases from −20 to 20 V. Figure 4: Electrical characterization of the cloned (7, 6) SWCNTs. ( a ) Schematic and ( b ) an SEM image (with artificial colour) of a back-gated (7, 6) nanotube transistor. The device consists of an individual (7, 6) nanotube, with L =4 μm and 50 nm thick SiO 2 gate dielectric. Scale bar, 5 μm for b . ( c ) Transfer characteristics ( I D – V G ) of the transistor measured at various V D biases. Inset, transfer characteristics plotted in semi-logarithm scale with V D =1 V. ( d ) Output ( I D – V D ) characteristics of the same device measured at various V G biases from −20 to 20 V. Full size image The transfer characteristics ( I D – V G ) measured at various V D biases, shown in Fig. 4c , clearly indicate that the device is made of a semiconducting nanotube. This is consistent with the (7, 6) chirality. Moreover, this nanotube delivered a respectable on-current of 5.4 μA at V D =1 V and V G =−15 V, which corresponds to~6 mA μm −1 when normalized by the nanotube diameter 0.89 nm. The maximum transconductance measured at V D =1 V was further calculated to be 0.74 mS μm −1 ( Supplementary Fig. S10 ). The linear output ( I D – V D ) characteristics of the same device shown in Fig. 4d also indicated formation of ohmic contacts between the nanotube and the metal contacts. We measured a total of 17 such devices produced with individual cloned (7, 6) nanotubes and found that all of them exhibit similar semiconducting behaviour ( Supplementary Fig. S11 ). Similar electrical characteristics were also observed for transistors made from cloned (6, 5) nanotubes ( Supplementary Fig. S12 ). These electrical measurements further confirm that chirality-controlled cloning was achieved and, moreover, demonstrate the preservation of superior electrical properties in the cloned nanotubes. What is the mechanism of the VPE-based SWCNT cloning? In what follows, we attempt to provide a molecular model to explain the effect of annealing, SWCNT growth and chirality-dependent growth rate. We emphasize the tentative nature of this model and present it in the spirit of stimulating further exploration of the VPE-based SWCNT cloning. We find that annealing is a critical step for successful SWCNT cloning. The edges of purified SWCNT seeds are created by the sonication process for dispersion. Cavitation ruptures C–C bonds, most likely leading to oxidation of carbons at the cutting edges to form –COOH, or reconstruction of carbons at the edges to form 5- or 7-membered ring structures, making the edges not suitable for continued growth. Air oxidation and subsequent hydrogen and water treatment most likely remove these defective carbons and expose more reactive hydrogen-terminated sp 2 carbon edges for growth ( Fig. 5a ). 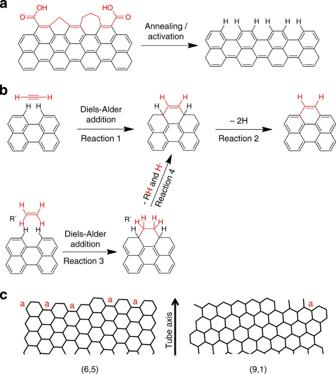Figure 5: Molecular mechanism of SWCNT cloning via VPE. (a) The effect of annealing. (b) Diels–Alder chemistry for the incorporation of C2H2and C2H4into an armchair site on the edge of a growing SWCNT seed. (c) Edge structures of unzipped ((6, 5) and (9, 1)) tubes. The red letteradenotes an armchair site on the edges. Figure 5: Molecular mechanism of SWCNT cloning via VPE. ( a ) The effect of annealing. ( b ) Diels–Alder chemistry for the incorporation of C 2 H 2 and C 2 H 4 into an armchair site on the edge of a growing SWCNT seed. ( c ) Edge structures of unzipped ((6, 5) and (9, 1)) tubes. The red letter a denotes an armchair site on the edges. Full size image What are the chemical reactions responsible for the observed nanotube growth in the absence of metal catalyst? VPE growth takes place at a high-enough temperature to thermally decompose carbon feed stock (methane or ethanol). There is a large body of literatures covering extensive studies on the pyrolysis process. To simplify our discussion and without loss of generality, we focus on the methane case [30] , [31] , [32] . Overall, pyrolysis of methane can be described by the reaction CH 4 →C (solid)+2H 2 . It starts with the rate-limiting radical generation reaction: CH 4 →CH 3 ·+H·. Following this is the formation of a variety of hydrocarbon species, including acetylene C 2 H 2 and ethylene C 2 H 4 . Indeed, we have detected C 2 H 2 and C 2 H 4 under our VPE growth condition using mass spectrometry, consistent with literature reports. Interestingly, also well-documented is the generation of high molecular weight species by the pyrolysis process, including polycyclic aromatic hydrocarbons, tar and coke. As a matter of fact, at temperatures above 850 °C, solid carbon and hydrogen are thermodynamically more favoured than any other hydrocarbon products [33] . Collectively, these results suggest that the chemistry between graphitic carbon structures and pyrolysis products is rich and may be exploited for SWCNT growth. In the context of these previous works, the essence of SWCNT cloning by VPE is to incorporate certain pyrolysis products into a graphitic carbon structure defined by the purified SWCNT seed. We propose that this is achieved by covalent addition of C 2 H 2 and C 2 H 4 at the SWCNT edge. More specifically, we propose that the chemistry between C 2 H 2 /C 2 H 4 and SWCNT edge follows the classic organic chemistry reaction for the generation of six-membered rings: Diels–Alder cycloaddition. As shown in Fig. 5b , acetylene C 2 H 2 can be incorporated into a site with armchair configuration through the Diels–Alder reaction (reaction 1), followed by a re-aromatization step (reaction 2). Similar reactions between C 2 H 2 and polycyclic aromatic hydrocarbons in organic solvents have been recently shown and proposed as the basis for metal-catalyst-free synthesis of SWCNTs by Fort et al . [34] , [35] Likewise, C 2 H 4 can also be incorporated into an armchair site through the Diels–Alder reaction (reaction 3). The C−C single bond created by reaction 3 can be converted into a double bond via a radical (CH 3 · or H·)-catalysed step (reaction 4). In both cases, the final product is a new six-membered sp 2 carbon ring built on the SWCNT edge. The whole process can be repeated at other existing or newly built armchair sites, resulting in elongation of the SWCNT with conservation of chirality defined by the seed. Growth termination may occur as a result of edge reactions with other reactive pyrolysis products. The Diels–Alder chemistry in the cloning mechanism requires the presence of armchair sites on the SWCNT edge. A natural consequence of this requirement is chirality-dependent growth rate. In general, for a ( n , m ) tube there are m armchair sites at the edge, and the rate of carbon incorporation should be proportional to m . The rate of tube length elongation R can be obtained after normalizing the rate of carbon incorporation by the tube circumference: Figure 5c illustrates the end edges of two semiconducting tubes of the same diameter (6, 5) and (9, 1), unzipped along the tube axis. According to the above analysis, (6, 5) tubes should grow five times faster than (9, 1). Precise rate measurement is challenging because of the short growth duration and non-synchronized initiation of growth [36] . Nevertheless, our preliminary data does show that (6, 5) tubes grow noticeable faster than (9, 1) tubes ( Supplementary Fig. S13 ). Interestingly, our conclusion of chirality-dependent SWCNT growth rate for VPE is similar to that of Ding et al . [37] for metal-catalysed SWCNT growth. This is because the armchair growth site in our model is equivalent to the ‘kink’ or ‘cosy corner’ in the model of Ding et al . [37] It should be noted that there are alternative mechanisms proposed for graphene edge growth without a metal catalyst, such as hydrogen atom-catalysed addition of C 2 H 2 (ref. 38 ). Further investigations are needed to develop quantitative growth rate measurement and to evaluate the role of different mechanisms in the VPE cloning process. In conclusion, we have demonstrated that chirality-controlled SWCNT growth can be achieved using catalyst-free VPE growth, which produces single-chirality, horizontally aligned nanotubes with significantly longer lengths than the as-purified seeds. Although this work only focused on the semiconducting (7, 6), (6, 5) and metallic (7, 7) nanotube species, we believe that the cloning process described here should be applicable to other semiconducting and metallic chiralities [26] . Our cloning method therefore opens up a possibility to study catalyst-free nanotube VPE growth mechanism as a function of chirality. With its versatility and reproducibility, the cloning technology platform should greatly benefit the device and circuit application of nanotubes. Moreover, future research on improving the cloning yield, density and precise positioning of the nanotube seeds could potentially lead to the long-dreamed, integrated functional ‘carbon-only’ electronic systems. VPE cloning of SWCNTs The chirality-pure (7, 6), (6, 5) and (7, 7) nanotube seeds were obtained using the DNA-based chromatographic purification [12] , [26] . Seed solutions with a concentration of ~0.5 μg ml −1 were drop-deposited onto quartz or Si/SiO 2 substrates and incubated for 30 min to 1 week, followed by gentle rinse with water and blow-dry. The samples were first annealed in a 2.54 cm (1 inch) tube furnace at 200 °C in air for 30 min. The temperature was then increased to 400 °C with the flow of 300 standard cubic centimetre per minute (sccm) hydrogen. Once the elevated temperature was reached, argon through a water bubbler kept at room temperature with a flow rate of 100 sccm was set to flow for 3 min. After the air and water vapour annealing and cooling down, VPE at 900 °C with either ethanol or methane as carbon feed source was used for nanotube growth. For both cases, 300 sccm of hydrogen was introduced during the temperature ramping-up process, which may terminate nanotube ends with hydrogen atoms. For the ethanol-based VPE growth, 300 sccm H 2 and 160 sccm Ar flowing through an ethanol bubbler kept at 0 °C was used; for the methane-based VPE growth, 2,000 sccm CH 4 and 300 sccm H 2 were used. For both cases, the growth was carried out for 15 min. We have conducted systematic explorations to define the stoichiometry for each species during the VPE cloning and to find the best recipe for cloning growth. In these experiments, ten samples with similar density of nanotube seeds were prepared and went through air and water vapour cleaning process together, and followed by cloning growth using ethanol as carbon source. We first investigated the effect of hydrogen concentration during cloning by varying the flow rate of hydrogen from 200 to 400 sccm, whereas keeping the flow rate of argon constant at 160 sccm. After VPE cloning, we used SEM to carefully examine the length, density and uniformity of cloned nanotubes. The results are shown in Supplementary Fig. S3a-d . Our results indicate that cloned nanotubes have the highest density when 300 sccm of H 2 and 160 sccm of Ar are used, whereas higher or lower flow rates of hydrogen reduce the yield of cloned nanotubes. Too high concentration of hydrogen is unfavourable, probably because it leads to hydrogenation and etching of nanotubes. On the other hand, too low concentration of hydrogen will likely produce less ordered carbon structures, such as amorphous carbon, which may hamper the nanotube growth, as suggested by literature reports [39] , [40] , [41] . We have also studied the effect of carbon concentration by keeping the hydrogen flow rate constant at 250 sccm and changing the argon flow rate from 200 to 108 sccm. The result is shown in Supplementary Fig. S3 e-h . The highest density was achieved when hydrogen flow rate is 250 sccm and argon flow rate is 128 sccm. We note a very interesting observation from these studies; the highest density occurred when the ratio between hydrogen and argon is around 2 (250/128=1.95 for the Supplementary Fig. S3g ; 300/160=1.88 for the Supplementary Figure S3c ). Characterization of cloned SWCNTs We used AFM (Digital Instrument Dimensional 3100, tapping mode), SEM (Hitachi, S4700) and Raman (Renishaw, with 633 and 532 nm lasers) to characterize VPE-grown SWCNTs. The integration time for the Raman spectra was 2 min. Device fabrication and electrical measurement We used electron beam lithography or photolithography to locate individual SWCNTs followed by e-beam evaporation and lift-off to form source and drain electrodes, which was made of 0.5 nm Ti and 50 nm Pd. The electrical measurement was conducted on Agilent 4156B. Certain commercial equipment, instruments or materials are identified in this paper to specify the experimental procedure adequately. Such identification is not intended to imply recommendation or endorsement by the National Institute of Standards and Technology, nor is it intended to imply that the materials or equipment identified are necessarily the best available for the purpose. How to cite this article: Liu, J. et al . Chirality-controlled synthesis of single-wall carbon nanotubes using vapour-phase epitaxy. Nat. Commun. 3:1199 doi: 10.1038/ncomms2205 (2012).